Exploiting multimode waveguides for pure fibre-based imaging There has been an immense drive in modern microscopy towards miniaturization and fibre-based technology. This has been necessitated by the need to access hostile or difficult environments in situ and in vivo . Strategies to date have included the use of specialist fibres and miniaturized scanning systems accompanied by ingenious microfabricated lenses. Here we present a novel approach for this field by utilizing disordered light within a standard multimode optical fibre for lensless microscopy and optical mode conversion. We demonstrate the modalities of bright- and dark-field imaging and scanning fluorescence microscopy at acquisition rates that allow observation of dynamic processes such as Brownian motion of mesoscopic particles. Furthermore, we show how such control can realize a new form of mode converter and generate various types of advanced light fields such as propagation-invariant beams and optical vortices. These may be useful for future fibre-based implementations of super-resolution or light-sheet microscopy. Complete control over the phase, amplitude and polarization of a light field may lead to startling results. In the last few years, we have seen the onset of a revolution in this area with particular regard to random media [1] , [2] , [3] . By performing a detailed analysis of the transmitted light field, we can adjust the input wavefront of a given light beam to control light propagation to unprecedented depths and to focus light at a given point in space despite deleterious scattering and in the presence of severe aberrations. At the heart of this method is the realization that the object has the form of a transmission matrix [3] , [4] that can be determined and utilized by feedback to a dynamic diffractive optical element to shape the incident wavefront for enhanced transmission and beam focusing. This area has already led to a new understanding of light propagation and the preliminary applications of imaging and micromanipulation at depth [2] , [4] , [5] , [6] . The concept of a disordered medium is broad and can embrace various photonics structures, particularly those that have the ability to simultaneously support multiple concurrent orthogonal modes of optical propagation. Multimode photonic waveguides are typically limited by modal dispersion restricting their application. Such dispersive effects lead typically to various forms of modal interference and 'unpredictable' output beam profiles such a speckle patterns. Separately, we are seeing a burgeoning need for imaging devices that offer observation in areas with typically very limited access and thus avoid the use of standard microscope platforms. In the biomedical arena, optical endoscopes aim to fulfil this need. While remarkable progress has been made in the miniaturization and spatial resolution enhancement of imaging modalities [7] , there is a need for further advancements. Endoscopes may be flexible or rigid in nature. Flexible endoscopes rely on image transfer through optical fibre bundles and are particularly important in observations through natural openings into organs [8] , [9] . These instruments, also known as fibrescopes, typically focus light through a miniaturized objective [10] or a gradient-index (GRIN) lens [11] that create an image on an input facet of a coherent fibre bundle, which subsequently acts as an image guide. Rigid endoscopes and borescopes are used in a number of clinical settings (for example, key-hole surgery) where natural openings are not available, as only instruments with rigid shafts can be controlled with sufficient precision in such cases (for example, neurosurgery [12] ). These instruments consist of a sequence of rod lenses periodically reconstructing the image along the optical axis and typically have cross-sections exceeding 1 mm in diameter. In this article, we demonstrate the transfer of imaging information along a fibre-based optical system. The image is neither separated into guiding channels in situ nor periodically repeated within an optical system but it is transmitted within a single-core multimode waveguide and reconstructed ex situ behind the fibre using the principles of digital holography. Crucially, by utilizing a multimode waveguide, the equivalent image information is relayed through a physical system with a cross-section one order of magnitude narrower than is possible with other available techniques [13] , [14] , [15] , [16] , [17] , [18] . The results we present offer several approaches to exploit multimode waveguides for imaging: we demonstrate a geometry for bright- and dark-field microscopy for monochromatic light as well as fluorescent imaging where the excitation wavelength is delivered in situ by the very same waveguide that also collects the fluorescence signal. Even though the geometries are based on different principles, our implementations allow image capture at very high frame rates in both cases, exceeding previously reported approaches by several orders of magnitude [19] . Furthermore, we show the controlled generation of complex light fields such as Laguerre–Gaussian modes, 'bottle' beams and propagation-invariant beams through a multimode fibre. This opens up prospects for fibre-based versions of techniques such as stimulated emission depletion microscopy (STED) or light sheet imaging. Based on the demonstrated results, we contend that our methodology paves the way for inexpensive 'lensless' imaging systems with diffraction-limited spatial resolution, minimal collateral damage and flexibility for use at various imaging depths or working distances. Bright- and dark-field imaging Within the geometry of a typical optical microscope, an infinity-corrected microscope objective performs a Fourier transform of the sample field into an intermediate plane. An inverse Fourier transform by a tube lens then forms an image that can be observed by the naked eye or captured by a camera. As the Fourier transform is very powerful and convenient for imaging, optical components such as lenses, focussing mirrors and objectives are carefully designed to perform in this manner. Adjusting the spatial frequency content of the sample field in the intermediate plane is at the heart of several important imaging techniques embedded within this Abbe formalism leading to concepts such as dark-field imaging or phase-contrast imaging, converting subtle but important phase changes to amplitude variations. The double Fourier transform is, however, not the only available choice when reconstructing a sample field across a remote plane. For monochromatic fields, in principle any pair of optical components providing an orthogonal transformation and a subsequent inverse transformation, respectively, can in fact be used. This leads us to the notion that even a multimode optical fibre, which entirely randomizes the propagating light, can be used for imaging in the same way as a microscope objective provided one can appropriately design an optical element that would render the inverse transform. To design such an element, one needs to analyse the overall field transformation that is performed by a particular multimode fibre together with other components of the geometry. This procedure, employing a spatial light modulator (SLM), was described previously in ref. 20 , and in Fig. 1 we show how we achieve such a calibration in our experimental geometry (see Methods for more details). The result of this calibration takes the form of a transformation matrix between orthogonal 'SLM modes'—with each mode comprising of reflected light from a square segment of the SLM chip—and 'sample modes' that refer to ideally focused light beams at a given distance behind the optical fibre. During the calibration, the SLM modes propagate from the SLM plane through the whole optical system (including the multimode fibre) into the sample, where they are recorded and analysed. 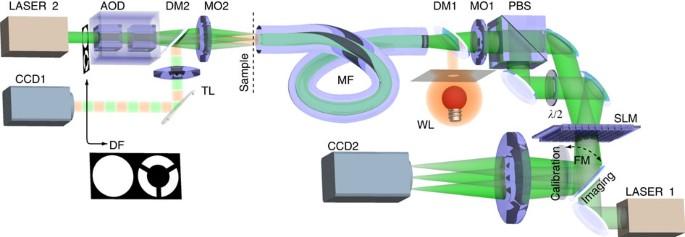Figure 1: Experimental geometry for the bright- and dark-field microscopy based on multimode fibre image transfer. During the calibration, light propagates from LASER 1 (operating at 1,064 nm) through the multimode optical fibre (MF, NA=0.22, 50 μm core diameter) onto the detector CCD1, imaging the fibre input facet (the sample plane). To couple into both polarization states, we split the light signal at the SLM into two pathways (superimposing different phase gratings20) that are later recombined on a polarizing beam splitter (PBS) before the resultant beam is coupled into the fibre by a microscope objective (MO1). LASER1 and CCD1 are only used for the calibration and subsequent verification of the imaging performance, and are not directly involved in the imaging process. A second laser (LASER 2) is used as an illumination signal during the imaging procedure. It is focused onto the sample plane by a second microscope objective (M02) and positioned in the plane by an AOD. In this manner, we can couple the light into the fibre from the opposite side in a controllable manner: we can generate focal spots (backwards propagating sample modes) or by rapid steering of the beam achieve arbitrary intensity patterns that simulate sample images. This way we can also generate a uniform spatially incoherent but monochromatic sample illumination, that we can then use for imaging of sample objects. Light from the sample plane propagates through the fibre onto the SLM chip where it is modified for imaging and consequently focused on CCD2 by a camera objective (CO). As the illuminating laser beam (LASER2) provides a larger NA than the multimode fibre, we can easily modify the system for dark-field imaging. Using an annular filter (DF) in a Fourier plane MO2, we restrict transmission to only those spatial frequencies exceeding the NA of the fibre. Such high-frequency components that directly propagate through an empty sample cannot be coupled into the fibre and thus do not contribute to the signal at CCD2. Only light redirected into the fibre by scattering from the object is coupled into the fibre thereby making the object visible. Figure 1: Experimental geometry for the bright- and dark-field microscopy based on multimode fibre image transfer. During the calibration, light propagates from LASER 1 (operating at 1,064 nm) through the multimode optical fibre (MF, NA=0.22, 50 μm core diameter) onto the detector CCD1, imaging the fibre input facet (the sample plane). To couple into both polarization states, we split the light signal at the SLM into two pathways (superimposing different phase gratings [20] ) that are later recombined on a polarizing beam splitter (PBS) before the resultant beam is coupled into the fibre by a microscope objective (MO1). LASER1 and CCD1 are only used for the calibration and subsequent verification of the imaging performance, and are not directly involved in the imaging process. A second laser (LASER 2) is used as an illumination signal during the imaging procedure. It is focused onto the sample plane by a second microscope objective (M02) and positioned in the plane by an AOD. In this manner, we can couple the light into the fibre from the opposite side in a controllable manner: we can generate focal spots (backwards propagating sample modes) or by rapid steering of the beam achieve arbitrary intensity patterns that simulate sample images. This way we can also generate a uniform spatially incoherent but monochromatic sample illumination, that we can then use for imaging of sample objects. Light from the sample plane propagates through the fibre onto the SLM chip where it is modified for imaging and consequently focused on CCD2 by a camera objective (CO). As the illuminating laser beam (LASER2) provides a larger NA than the multimode fibre, we can easily modify the system for dark-field imaging. Using an annular filter (DF) in a Fourier plane MO2, we restrict transmission to only those spatial frequencies exceeding the NA of the fibre. Such high-frequency components that directly propagate through an empty sample cannot be coupled into the fibre and thus do not contribute to the signal at CCD2. Only light redirected into the fibre by scattering from the object is coupled into the fibre thereby making the object visible. Full size image Such a calibration must be repeated for any substantial physical change to the spatial configuration, that is, fibre bends or loops. However, we have found that the calibration is tolerant to certain bending ( Supplementary Fig. S1 ) and in our settings the geometry can perform reproducibly without the need for recalibration for periods of weeks. After the calibration procedure, we reset the system for imaging: in this case we collect light from the sample, through the fibre onto the SLM where knowledge of the calibrated fibre allows us to perform imaging—simultaneous measurement of optical power within different locations of the sample—that is, carried by backwards propagating sample modes. For this purpose, the SLM carries an imaging hologram that we synthesize as a superposition of modulations corresponding to individual sample modes (see Fig. 2 and Methods). 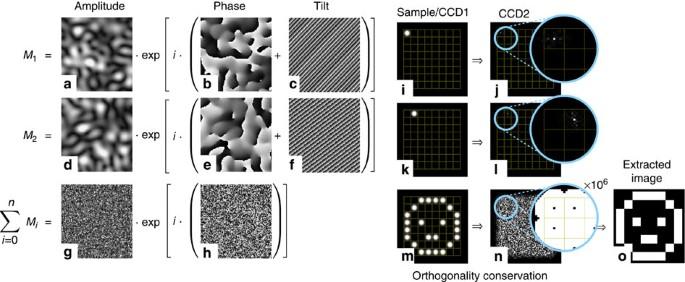Figure 2: Synthesis of imaging holograms. Panelsa–oare computer simulations to outline the method. (a–c,d–f) Examples of two modulations that, when applied on the SLM while LASER 2 is focussed onto the corresponding locations in the sample plane (i,k), generate proportional signals on specific pixels at the CCD2 (j,l). (g,h) The imaging hologram is a superposition of a number of such modulations, and when applied on the SLM the system can achieve imaging of a number of sample pointsmonto series of specific CCD pixels simultaneously (n,o), in principle with no crosstalk between individual points owing to the conservation of orthogonality within the system. The resulting imageois reconstructed from these 'active' pixels. Blue circles inj,landnshow expanded areas of a CCD plane. The signal in the expansion circle of panelnis scaled by six orders of magnitude beyond the point of saturation and still the isolated 'active' pixels corresponding to the dark sample locations give no signal owing to orthogonality conservation. Figure 2: Synthesis of imaging holograms. Panels a – o are computer simulations to outline the method. ( a – c,d – f ) Examples of two modulations that, when applied on the SLM while LASER 2 is focussed onto the corresponding locations in the sample plane ( i , k ), generate proportional signals on specific pixels at the CCD2 ( j , l ). ( g , h ) The imaging hologram is a superposition of a number of such modulations, and when applied on the SLM the system can achieve imaging of a number of sample points m onto series of specific CCD pixels simultaneously ( n , o ), in principle with no crosstalk between individual points owing to the conservation of orthogonality within the system. The resulting image o is reconstructed from these 'active' pixels. Blue circles in j , l and n show expanded areas of a CCD plane. The signal in the expansion circle of panel n is scaled by six orders of magnitude beyond the point of saturation and still the isolated 'active' pixels corresponding to the dark sample locations give no signal owing to orthogonality conservation. Full size image With the pixel resolution of the used detector CCD2 and the SLM, we were able to simultaneously image 144 sample modes (12×12) at a rate restricted solely by the CCD (200 Hz). The resultant pixel resolution, however, does not provide sufficient sampling of the field. Therefore, we used nine different imaging holograms sequentially applied by the SLM, to increase the pixel resolution to 36×36 pixels at the expense of the frame rate. To reconstruct one sample image, we need to combine nine different frames from the detector CCD2 obtained for nine different imaging holograms sequentially applied on the SLM operating at 100 Hz. In the optimal case, one would expect that the frame rate is reduced to 1/9 of the SLM rate, that is, 11 Hz; however, due to synchronization issues between CCD2, the SLM and the controlling computer the attainable frame rate was further reduced to 5.4 Hz. With these settings, the system can image any field along the sample plane with more than ×4 higher pixel resolution than the number of modes allowed to propagate within the system. Hence, the sampling rate exceeds the Nyquist frequency. A further increase in the pixel resolution would increase the signal/noise ratio, but would not influence the image sharpness. The numerical aperture (NA) dictates the maximal spatial resolution of our fibre imaging system. There are, however, no restrictions in performing the calibration and recording images at any axial distance behind the fibre. As we alter the distance from the fibre facet, a trade-off occurs: we lose spatial resolution but obtain a wider field of view. As the total number of modes allowed to propagate in the fibre is fixed, the final information content of the image remains unchanged regardless of the distance from the fibre facet where we image. More details on this aspect are given in Supplementary Fig. S2 . Throughout our experiments, the imaging plane was set to ≈30 μm behind the fibre facet to allow a convenient working distance but still achieve maximal spatial resolution in imaging. The only exception to this was the imaging of laser-scanning fields ( Fig. 3a–f ) where the imaging plane was set directly onto the fibre facet. This is to allow additional imaging pathway to be used for direct observation of the sample field retro-reflected at the fibre facet by the means of standard microscopy, giving a further confirmation of the performance of our system. 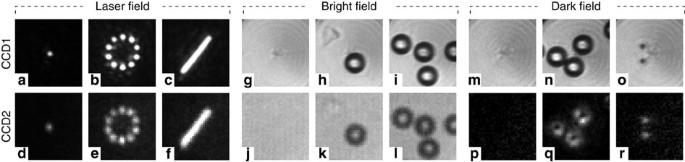Figure 3: Bright- and dark-field microscopy based upon multimode fibre image transfer. The top row shows images obtained by direct imaging of sample (CCD1, seeFig. 5) whereas the bottom row presents the images reconstructed from the randomized output light at the other end of the fibre and detected by CCD2 (Fig. 5). (a–f) Imaging of laser fields generated by scanning a laser beam focus along the input fibre facet by an AOD. (g–l) Bright-field images of empty sample (g,j) and 10-μm polymer particles in a water solution (h,iandk,l). (m–r) Dark-field images of empty sample (m,p) and polymer particles of 10 μm (n,q) and 1.8 μm (o,r) in diameter, respectively. Figure 3: Bright- and dark-field microscopy based upon multimode fibre image transfer. The top row shows images obtained by direct imaging of sample (CCD1, see Fig. 5 ) whereas the bottom row presents the images reconstructed from the randomized output light at the other end of the fibre and detected by CCD2 ( Fig. 5 ). ( a – f ) Imaging of laser fields generated by scanning a laser beam focus along the input fibre facet by an AOD. ( g – l ) Bright-field images of empty sample ( g , j ) and 10-μm polymer particles in a water solution ( h , i and k , l ). ( m – r ) Dark-field images of empty sample ( m , p ) and polymer particles of 10 μm ( n , q ) and 1.8 μm ( o , r ) in diameter, respectively. Full size image The performance of the system is presented in Fig. 3 for the case of acousto-optic deflector (AOD)-generated (scanned) laser images ( Fig. 3a–f ), bright-field images ( Fig. 3g–l , the AOD provides uniform illumination) and the dark-field alternative ( Fig. 3m–r ). Individual approaches are also demonstrated in Supplementary Movies 1, 2 and 3 . The presence of noise can be observed in figures Fig. 3b,e . There are several contributions to this unwanted signal including CCD noise and crosstalk between imaging points; however, their magnitude did not exceed −30 dB. Fluorescent imaging Both the presented bright- and dark-field imaging methods rely on the monochromatic nature of the light propagating in the system. The requirements on the spectral purity of the illumination light are high (a frequency bandwidth of no more than a few gigahertz is required for our bright-field geometry, see Supplementary Discussion ). However, when fluorescent imaging is considered, the fluorescence light is typically emitted with a very broad spectrum. Such a signal could not be analysed behind the fibre using the bright-field imaging technique explained earlier without major power losses while filtering out a single wavelength. On the other hand, the excitation wavelength can have a very narrow bandwidth. Using the knowledge of the fibre field transformation, the excitation light can be delivered through the fibre sequentially to distinct points across the sample plane (sample modes) to excite a fluorescent dye within the corresponding spatial regions, analogously to an epi-fluorescence laser-scanning microscope. The total intensity signal of fluorescent emission originating from each of these diffraction-limited sample locations may be collected through the very same fibre by an appropriate detector [19] without any requirements upon spectral purity. The resulting fluorescent sample image is then reconstructed from an array of these intensity measurements assigned to corresponding sample points. Reconfiguring the SLM for measurement of each of the sample points sequentially is straightforward but even with the fast SLM we use in our geometry (Boulder Nonlinear Systems) we only reach rates of the order of 100 Hz. An image containing 1,000 data points would thus be scanned in the relatively long interval of 10 s. This, however, compares favourably with a related approach recently published [19] , where an image of 3,600 points was obtained within an interval of ∼ 3 min. In contrast to the SLM, the technology of the AOD can be employed to redirect a laser beam with very fast rates, but does not lend itself to more complex beam shaping owing to the absence of facile phase modulation. Both technologies were developed in parallel in the branch of optical manipulation, but only recently were they combined into a more powerful tandem system that immediately manifested itself as an extraordinary optical tool allowing fast and complex beam shaping [21] , [22] , [23] . We employ this assembly to provide fast scanning (40 kHz) of a single focal spot behind the fibre output to provide fluorescence excitation. A fast and sensitive detector synchronized with the AOD scanning collects the fluorescent emission delivered backwards by the optical fibre ( Fig. 4 ). We show that this leads to an enhancement of the imaging speed by two orders of magnitude. Imaging holograms are also in this case generated as a superposition of a number of modulations corresponding to selected sample modes (see Fig. 5 ). The Methods section presents more details about the experimental geometry and the synthesis of imaging holograms. 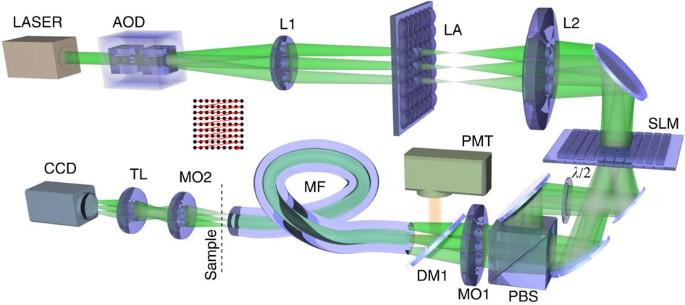Figure 4: Experimental geometry for the fluorescent microscopy based on multimode fibre image transfer. The appropriate selection of lenses L1 and L2 and a lenslet array LA provides expansion and collimation of the laser beam on the SLM. During calibration, the AOD deflects the initial laser beam onto a central segment of the lenslet array and these settings are kept unchanged during the calibration measurement. Similarly as in the case of bright-/dark-field geometry, using a polarization beam splitter PBS and a half-wave plate λ/2 the light is coupled into the fibre (by microscope objective MO1) in both polarization states to achieve maximal efficiency. The signal leaving the fibre is imaged onto the CCD by a telescope (MO2 and TL). Once the calibration is accomplished, we reset the system for imaging. In this case, the AOD periodically alternates the alignment of the beam onto different segments of the LA that changes the angle of the incidence onto the SLM. The imaging hologram applied to the SLM acts in such a way that for every angle of incidence of the laser beam the light behind the fibre forms an optimally focussed beam at different locations across the sample plane. This provides a rapid scanning of the focused excitation beam. Fluorescence emission light from illuminated objects is collected by the fibre, separated from the excitation pathway using a dichroic mirror DM1 and detected by photomultiplier PMT. Figure 4: Experimental geometry for the fluorescent microscopy based on multimode fibre image transfer. The appropriate selection of lenses L1 and L2 and a lenslet array LA provides expansion and collimation of the laser beam on the SLM. During calibration, the AOD deflects the initial laser beam onto a central segment of the lenslet array and these settings are kept unchanged during the calibration measurement. Similarly as in the case of bright-/dark-field geometry, using a polarization beam splitter PBS and a half-wave plate λ/2 the light is coupled into the fibre (by microscope objective MO1) in both polarization states to achieve maximal efficiency. The signal leaving the fibre is imaged onto the CCD by a telescope (MO2 and TL). Once the calibration is accomplished, we reset the system for imaging. In this case, the AOD periodically alternates the alignment of the beam onto different segments of the LA that changes the angle of the incidence onto the SLM. The imaging hologram applied to the SLM acts in such a way that for every angle of incidence of the laser beam the light behind the fibre forms an optimally focussed beam at different locations across the sample plane. This provides a rapid scanning of the focused excitation beam. Fluorescence emission light from illuminated objects is collected by the fibre, separated from the excitation pathway using a dichroic mirror DM1 and detected by photomultiplier PMT. 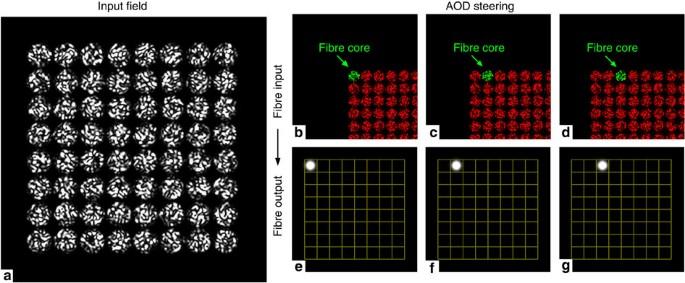Figure 5: Matrix of generating fields at the fibre input. These images are computer simulations of the resulting optical field at the plane of the input fibre facet and the resulting sample modes (ideally focussed beams) corresponding to different AOD settings. (a) The SLM generates a matrix of optical fields corresponding to a series of sample modes. (b–d) The AOD sequentially aligns individual segments on the fibre core, that results in scanning of the focussed beam along the sample plane (e–g). Full size image Figure 5: Matrix of generating fields at the fibre input. These images are computer simulations of the resulting optical field at the plane of the input fibre facet and the resulting sample modes (ideally focussed beams) corresponding to different AOD settings. ( a ) The SLM generates a matrix of optical fields corresponding to a series of sample modes. ( b – d ) The AOD sequentially aligns individual segments on the fibre core, that results in scanning of the focussed beam along the sample plane ( e – g ). Full size image Within our geometry, for a single imaging hologram applied on the SLM, we can reach up to 11×11 image points, that, analogously to the bright-field imaging, does not provide sufficient sampling. Therefore, we synthesize a number of different imaging holograms to be sequentially exposed by the SLM. Also, owing to a number of synchronization issues between the controlling computer, SLM, AOD and photomultiplier (PMT), we could only operate the system at about half the rate corresponding to the limitation by the slowest component (SLM). The performance of the fluorescent imaging is presented in Fig. 6 and Supplementary Movie 4 for varying resolutions and corresponding frame rates. 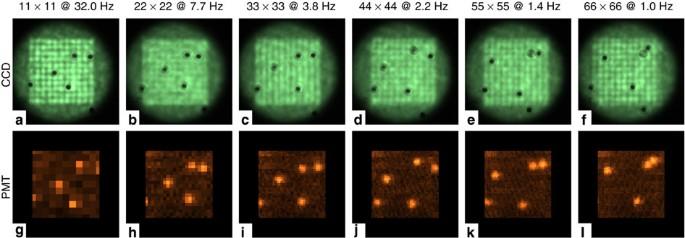Figure 6: Multimode fibre-based fluorescence microscopy. The sample contains fluorescent polymer particles having 2 μm in diameter. The top row (a–f) shows images sample volume directly imaged onto a CCD detector (seeFig. 6). Excitation signal in the form of 11×11 matrix of focal points is clearly visible. The bottom row (g–l) are images reconstructed from the fluorescence signal detected by a PMT (Fig. 6) behind the optical fibre. Each column shows the imaging performance for different resolution and frame rates. (a,g) Imaging for one static hologram at the SLM giving image resolution of 11×11 data points with 32 frames per second. (b,h) The SLM cycles between four different holograms to increase the resolution to 22×22 data points at the expense of frame rate, reduced to 7.7 Hz. (c,i) The SLM cycles between nine different holograms leading to 33×33 data points and frame rate of 3.8 Hz. (d,j) The SLM cycles between 16 holograms leading to 44×44 data points and frame rate of 2.2 Hz. (e,k) The SLM cycles between 25 holograms leading to 55×55 data points and frame rate of 1.4 Hz. (f,l) The SLM cycles between 36 holograms leading to 66×66 data points and frame rate of 1.0 Hz. Figure 6: Multimode fibre-based fluorescence microscopy. The sample contains fluorescent polymer particles having 2 μm in diameter. The top row ( a – f ) shows images sample volume directly imaged onto a CCD detector (see Fig. 6 ). Excitation signal in the form of 11×11 matrix of focal points is clearly visible. The bottom row ( g – l ) are images reconstructed from the fluorescence signal detected by a PMT ( Fig. 6 ) behind the optical fibre. Each column shows the imaging performance for different resolution and frame rates. ( a , g ) Imaging for one static hologram at the SLM giving image resolution of 11×11 data points with 32 frames per second. ( b , h ) The SLM cycles between four different holograms to increase the resolution to 22×22 data points at the expense of frame rate, reduced to 7.7 Hz. ( c , i ) The SLM cycles between nine different holograms leading to 33×33 data points and frame rate of 3.8 Hz. ( d , j ) The SLM cycles between 16 holograms leading to 44×44 data points and frame rate of 2.2 Hz. ( e , k ) The SLM cycles between 25 holograms leading to 55×55 data points and frame rate of 1.4 Hz. ( f , l ) The SLM cycles between 36 holograms leading to 66×66 data points and frame rate of 1.0 Hz. Full size image Advanced beam shaping for complex imaging methods As we now progress to show, exploiting the disorder in multimode fibres may yield a number of non-zero-order light modes that are essential for more complex applications including super-resolution imaging techniques. The multimode fibre in this instance acts akin to a mode converter. As discussed, for example, in ref. 24 , the light propagating within the fibre is not randomized with loss of all parameter knowledge. A very important aspect in the randomization process is utilized; light coupled into the fibre with a specific propagation constant k z (axial component of the k vector) will leave the fibre output with this quantity conserved ( Fig. 7a ). The coupling between radial modes is described by a coupling coefficient, that depends on the fibre quality and length, and is typically very low. Hence in our geometry, SLM modes located within a specific annular zone at the SLM plane will form an orthogonal subspace not interacting (significantly) with modes in other zones. This means that each azimuthally independent spectral modulation of the optical field at the fibre input will have an identical influence on the spatial spectrum of the output field. In other words, for azimuthally independent spectral modulations, the multimode fibre behaves as a Fourier space device. This substantially broadens the spectrum of light shapes that we can generate within the sample. Adding a constant phase shift of π to the appropriately sized central circular zone of the original phase modulation ( Fig. 7b ) converts the initial ideally focussed sample mode to a 'bottle' beam [25] , [26] . Its lateral and azimuthally averaged longitudinal cross-sections are presented in Fig. 7e,f . This might, for example, allow the realization STED microscopy deep within turbid media by employing our fibre-based system at two different wavelengths. Similarly, annular filtering [27] ( Fig. 7c ) transforms the sample mode to a zero-order Bessel beam ( Fig. 7g,h ) that can be used for a broad spectrum of optical manipulation techniques. If this beam is rapidly steered along one direction (using a tandem SLM-AOD system), it will generate an ideal field for light-sheet microscopy (LSM) [28] . This may be delivered within turbid environments by the fibre directly to the imaging plane without scattering losses and randomization. A further very important demonstration is that of a quadratic radial phase modulation ( Fig. 7d ), that causes an axial shift of the sample mode (or any other beam type). This way one can refocus upon another axial plane when imaging without the need to recalibrate the system. Longitudinal cross-sections of a sample mode axially positioned into several different sample depths are shown in Fig. 7i . Other applications of this powerful feature might involve manipulation of the NA of the sample modes (that we employed for fluorescent imaging) or in combination with appropriate illumination, fibre-based phase-contrast microscopy. 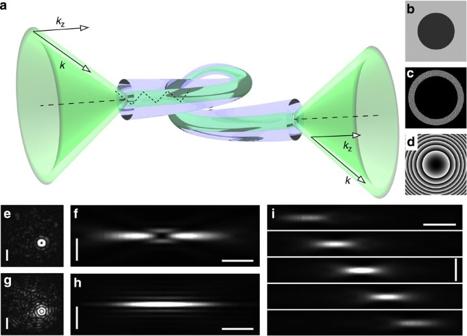Figure 7: Shaping of output modes by azimuthally independent modulations. (a) Conservation of the propagation constant: light coupled into the fibre with a specific propagation constantkzwill leave the fibre with this quantity unchanged. (b) Holographic modulation to convert a sample mode into a 'bottle' beam. (c) Annular filtering of the sample mode leads to generation of a Bessel beam. (d) Quadratic radial phase modulation (defocus) shifts the sample mode axially. Panelsf,handiare azimuthally averaged projections of three-dimensional data stacks obtained from a series of CCD frames (e,g) obtained at different axial distances behind the fibre. For all the panelse–i, the vertical scale bars correspond to distance of 10 μm while horizontal ones correspond to 50 μm. Figure 7: Shaping of output modes by azimuthally independent modulations. ( a ) Conservation of the propagation constant: light coupled into the fibre with a specific propagation constant k z will leave the fibre with this quantity unchanged. ( b ) Holographic modulation to convert a sample mode into a 'bottle' beam. ( c ) Annular filtering of the sample mode leads to generation of a Bessel beam. ( d ) Quadratic radial phase modulation (defocus) shifts the sample mode axially. Panels f , h and i are azimuthally averaged projections of three-dimensional data stacks obtained from a series of CCD frames ( e , g ) obtained at different axial distances behind the fibre. For all the panels e – i , the vertical scale bars correspond to distance of 10 μm while horizontal ones correspond to 50 μm. Full size image The versatility of the method is seen from the fact that any other beam shape required for a specific application can be formed by combining sample modes with an appropriate amplitude, phase and polarization [20] . A key illustrative example is the generation of optical vortices, that we create from a number of modes positioned along a circle of an adequate radius while gradually shifting the phase of the sample modes accordingly to the required topological charge (integer number of 2 π phase elevations along the circumference, see Fig. 8a ). A sequence of optical vortices with topological charge from an interval of l ∈ −3,3 in integer steps is presented in Fig. 8b , together with interferograms of vortices of l =±1 with a plane wave while gradually increasing a phase delay between them, thus confirming the helicity of the resulting wavefront, typical for these fields ( Fig. 8c,d ). 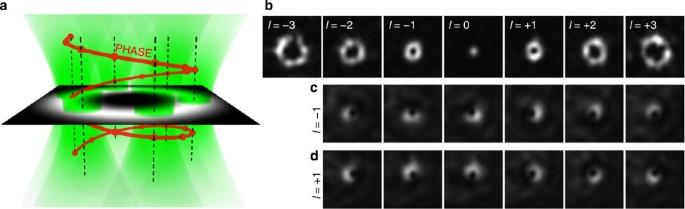Figure 8: Generation of non-zero-order modes. (a) Any optical field (within the accessible field of view and range of spatial frequencies supported by the optical fibre) can be expressed as a superposition of the output modes. For the specific case of optical vortices, we distribute a series of output modes along a circle of an appropriate diameter and offset their phases accordingly to the required topological shape of the final wavefront. (b) Experimentally generated optical vortices with varying topological charge. (c,d) Interferograms ofl=±1 vortices with a plane wave for six different phase shifts of the plane wave covering an interval of0,2π. Rotation of the phase singularity (dark spot) along the vortex circumference reveals its helical wavefront together with its handedness. Figure 8: Generation of non-zero-order modes. ( a ) Any optical field (within the accessible field of view and range of spatial frequencies supported by the optical fibre) can be expressed as a superposition of the output modes. For the specific case of optical vortices, we distribute a series of output modes along a circle of an appropriate diameter and offset their phases accordingly to the required topological shape of the final wavefront. ( b ) Experimentally generated optical vortices with varying topological charge. ( c , d ) Interferograms of l =±1 vortices with a plane wave for six different phase shifts of the plane wave covering an interval of 0,2π . Rotation of the phase singularity (dark spot) along the vortex circumference reveals its helical wavefront together with its handedness. Full size image Randomized light fields open up new forms of imaging. We have shown that the use of a simple step-index multimode optical fibre provides startling new ways to form bright- and dark-field images as well as form a range of sculptured advanced light beams. Coherent light propagating through such a waveguide is randomized but the image information is not lost and can be decoded once the overall system transformation is measured. As the sample plane can be defined at any distance from the fibre facet, we eliminate the need for complex or elaborate focusing optics (for example, miniaturized objectives, GRIN lenses) and instead reconfigure the system dynamically at the SLM to image different axial planes. Our experiments were performed in the vicinity of the fibre to achieve the highest spatial resolution, but one can select another remote plane to gain an increased field of view. In future, this could allow a 'zooming' ability of the system providing multiple calibrations at a series of different axial sample planes. Using multimode fibres also allows for a reduction in the size of the image guide by an order of magnitude compared with currently available fibre bundles. We have presented a geometry for bright-field imaging, where spatially incoherent, but monochromatic, light illuminating the sample plane was holographically converted after propagation through the multimode fibre into the form of a sample image. Even though this technique presently requires trans-illumination of the sample, an appropriate light signal can be delivered into the image plane through very thick and highly scattering environments. In the case of dark-field imaging, the sample illumination is restricted to a certain range of spatial frequencies, that is not achievable through thick scattering samples owing to strong randomization. This could, however, be applied using multilayer imaging fibres providing the illumination in an annular region surrounding the central imaging core. The second geometry presented employed a static hologram to allow rapid scanning of an excitation beam into the sample through the multimode fibre core. The same fibre also collected fluorescent signal from sample objects and delivered it to a detector. Both geometries were successfully tested by imaging polymer particles in close proximity to the fibre facet, with sufficient pixel resolution for sampling of the fibre core area and imaging speeds approaching video rate. Presently, after the system calibration is accomplished, the fibre must be kept static for the duration of the experiment. Further engineering may, however, substantially miniaturize the optical pathways that could lead to the introduction of compact endoscopic hand-held devices for clinical, scientific or industrial applications where rod-lens-based rigid endoscopes currently dominate. As shown in Supplementary Fig. S1 , some flexibility of the fibre can be tolerated; however, for larger changes in its configuration (bending or looping), the system has to be calibrated sequentially for every configuration required. The geometries were built with standard commercially available components, leading to a relatively limited frame rate and pixel resolution, and these could also be vastly improved in the future. To the best of our knowledge, this technology represents the narrowest possible image guiding system based on light propagation. The spectrum of applications is very broad, with particular importance for fibre-based 'lensless' microscopes and minimally invasive rigid endoscopes. Future work will explore improvements in pixel resolution and imaging rates, but also the employment of alternative waveguides, especially GRIN multimode optical fibres, that could minimize the requirement for high spectral purity of the laser source and possibly allow for multiphoton excitation. We will explore application of this technology for other advanced types of microscopy (STED and LSM) and investigate the use of sculptured light beams, such as optical eigenmodes [29] that can further be exploited for imaging [30] . Other applications might include visualization of complex systems such as quantum gases in optical lattices [31] . Exploring the light randomization process within the fibre and the so termed 'memory effect' [32] , [33] may lead to a greater degree of tolerance of fluctuations in the fibre arrangement. If we can overcome this to a greater extent, this may allow for additional flexibility of the fibre waveguide during imaging. Bright- and dark-field imaging system This section explains the functionality of our experimental geometry that we use for the bright- and the dark-field imaging. As discussed earlier, the necessary task to be accomplished before the system can act as an imaging device is to quantify the way the light propagates within the particular experimental geometry, that is, measure the transformation matrix of the system, and based on this result design an imaging hologram efficiently inverting this transformation to reconstruct an image of the sample field. The method we use for this purpose will henceforth be referred to as 'the calibration' and was described earlier [20] . In the following text, we will briefly revisit its foundations. Figure 1 presents a simplified scheme of our experimental geometry. The calibration technique is based upon a field decomposition into a series of orthogonal optical modes defined in the plane of a SLM and further sequentially analysed behind the randomizing optical system by interference with a reference signal [1] , [2] , [3] . We remark that alternative algorithms based on different strategies (for example, phase-only direct-search approach [34] ) were recently identified. For optimal efficiency, light must be coupled into the fibre in both polarization states and, importantly, the orthogonality of output modes [20] must be maintained. It transpires that this is particularly essential for optimal performance in the case of bright-field imaging (see Supplementary Figs S3–S5 and Supplementary Discussion ). As explained previously [20] , we use an external reference via a separate optical pathway to get the highest efficiency for all output modes. Once the calibration is finished, we obtain a complete knowledge of the optical transformation between the SLM plane and the sample plane (fibre facet), where we can concentrate the light into a series of ideally focussed beams that we term 'sample modes'. It is not possible to achieve an inverse transform, that would form a compact sample image at the CCD detector, solely with the use of one static planar hologram. However, at the expense of optical power, the sample image can be reconstructed from values measured by a series of discrete pixels regularly distributed across the CCD 2 matrix ( Supplementary Discussion provides more details on these principles). As explained in Fig. 2 , the imaging hologram is generated as a complex superposition of a number of modulations, generating individual sample modes ( M 1 ... M n ), each of these being subject to a specific blazed phase grating ( Fig. 2a–f ). Each of the modulations M 1 ... M n when applied independently provide a scalar product between the sample field with a specific sample mode, that is, they yield a measure of the intensity of a particular sample point regardless of the distribution of the light elsewhere. When the complete hologram ( Fig. 2g,h ) is applied by the SLM, the light field from the image propagating from the fibre is split and deflected to separate regions along the CCD plane where, in each region, a single isolated pixel simultaneously provides a measurement of the intensity of a specific sample point. In this way, we efficiently invert the field transformation of the multimode fibre using a single static diffractive element that thus acts analogously to a tube lens in a Fourier imaging system. Note that this approach complements that developed by Popoff et al . [4] , where the image was numerically extracted from a record of the complex speckle distributions that result after traversing an opaque medium using knowledge of the transmission matrix of the medium. Further details about the experimental geometry and the imaging hologram synthesis may be found in Supplementary Fig. S6 and Supplementary Discussion . To allow direct visualization within the sample during testing of this approach, we introduced a white-light illumination of the sample through the fibre, which was subsequently detected at CCD1. Fluorescent imaging system Our geometry is presented in Fig. 4 . To excite the red fluorescent dye (Firefli Red), we reconfigured the system to operate at a wavelength of 532 nm. Analogously to the previous case, after the calibration procedure, we generate the imaging hologram as a complex superposition of modulations corresponding to a single sample mode, again each amended by specific phase tilt. If applied on the uniformly illuminated SLM, the resulting light distribution at the input fibre facet forms a matrix of non-overlapping optical landscapes—generating fields—each confined within an area corresponding to the size of the fibre core ( Fig. 5a ). Each of these fields generates a specific sample mode if coupled into the fibre ( Fig. 5b–g ). If the beam propagating onto the SLM is steered between discrete sets of incident angles, individual generating fields are aligned into the fibre resulting in the formation of sample modes sequentially generated at specific locations across the sample plane ( Fig. 5b–g ). Effectively, for these incident angles, the whole system of SLM, relay optics and multimode fibre operate as a Fourier component (microscope objective). In this configuration, we can deploy a very fast AOD to provide the steering and the system works analogously to a laser-scanning microscope. The range of deflection angles the AOD can provide, however, does not fully cover our requirements. As for this application we do not need the full spectrum of deflection angles, but only a series of discrete values, we can efficiently magnify the deflection range by combining the AOD with a lenslet array (marked LA on Fig. 4 ). This way we can steer the focussed beam within the sample at very high rates that are constrained only by the AOD rise/fall times. The fluorescence signal is registered at a PMT for every AOD configuration at rates of 40 kHz. At the excitation wavelength, the number of modes propagating in the system is four times larger than in the case of bright-field imaging [35] . Even though the SLM used features sufficient for pixel resolution to provide the corresponding number of modes for orthogonal fibre transformation, it could only form a very limited number of generating fields along the input plane that would later significantly slow down the imaging. Therefore, we reduced the NA of the light coupled into the fibre by 33%, which allowed us to accommodate up to 11×11 generating fields across the input plane. This NA reduction limited the number of orthogonal output modes by more than 50% and increased their diameter to 2.21 μm. However, as we can utilize the role of azimuthally independent modulations (discussed later), this did not compromise the orthogonality of the transformation (crosstalk between imaging points), but solely reduced the spatial resolution of the imaging owing to increased size of sample modes. Further details about the experimental geometry may be found in Supplementary Fig. S7 . How to cite this article: Čižmár, T. & Dholakia, K. Exploiting multimode waveguides for pure fibre-based imaging. Nat. Commun. 3:1027 doi: 10.1038/ncomms2024 (2012).